DNA replication timing and higher-order nuclear organization determine single-nucleotide substitution patterns in cancer genomes Single-nucleotide substitutions are a defining characteristic of cancer genomes. Many single-nucleotide substitutions in cancer genomes arise because of errors in DNA replication, which is spatio-temporally stratified. Here we propose that DNA replication patterns help shape the mutational landscapes of normal and cancer genomes. Using data on five fully sequenced cancer types and two personal genomes, we determined that the frequency of intergenic single-nucleotide substitution is significantly higher in late DNA replication timing regions, even after controlling for a number of genomic features. Furthermore, some substitution signatures are more frequent in certain DNA replication timing zones. Finally, integrating data on higher-order nuclear organization, we found that genomic regions in close spatial proximity to late-replicating domains display similar mutation spectra as the late-replicating regions themselves. These data suggest that DNA replication timing together with higher-order genomic organization contribute to the patterns of single-nucleotide substitution in normal and cancer genomes. Human cancer genomes exhibit complex mutational landscapes, often characterized by a large number of single-nucleotide substitutions (SNS) found throughout the genome [1] , [2] , [3] . The patterns of SNS have been shown to depend on the type of cancer, the number of cell divisions leading to the initiation and progression of the tumour and tissue-specific patterns of driver events in cancer [4] , [5] , [6] , [7] . Mutation rates also vary according to different genomic features such as GC content, recombination rate, CpG islands and others [8] , [9] , [10] . Recent advances in genomic profiling methods have enabled the characterization of the spatial arrangement of genomic material within inter-phase nuclei [11] , [12] . The use of such databases has enabled an unprecedented mapping of genomic regions not only relative to each other but also with regard to different higher-order structures within individual cell types [11] , [13] , [14] . Furthermore, the temporal order of DNA replication in human cells displays marked variability across genomic regions, in that some areas are replicated early, whereas others are replicated late during S phase [15] , [16] , [17] . To date, such data has been used to investigate evolutionary divergence between species and human nucleotide diversity, showing that late-replicating regions display larger point mutation rates than early-replicating regions [18] . It was also recently elucidated that genomic regions of similar replication timing are clustered spatially in the nucleus, that the two boundaries of somatic copy number alterations (SCNAs) in cancer genomes tend to be found in regions with the same replication timing and that regions replicated early and late display distinct patterns of frequencies of SCNA boundaries, SCNA size and a preference for deletions over insertions [19] . For example, deletions are generally more frequent than amplifications in late as compared with early replication timing zones. Recently available genome-wide sequencing data have enabled us to investigate the patterns of SNS in different temporal phases and spatial compartments during the DNA replication process. Several studies have illustrated associations between mutation frequencies and other genetic and epigenetic factors [20] , [21] , [22] . Woo et al . [20] utilized information on selection and DNA replication timing to study the local variation of mutation frequencies, whereas Schuster-Bockler et al . [21] and the The Cancer Genome Atlas (TCGA) lung cancer consortium [21] , [22] proposed a multivariate analysis approach to investigate epigenetic markers using data from different cell types. Here we investigated the patterns of SNS across the genome by using replication timing data conserved across several cell lines based on data from Hansen et al . [23] and regions not under strong selection pressure [24] . We then comprehensively catalogued individual mutation signatures in these constant late and early replication timing zones. Finally, we utilized information on higher-order chromatin interactions between genomic material to demonstrate the coordinative effects between replication timing and nuclear architecture on the mutational landscape of cancer genomes. 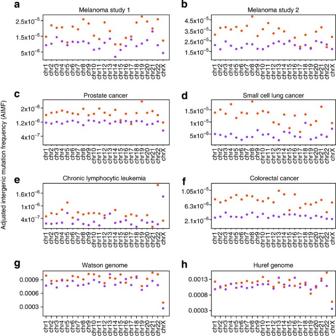Figure 1: Effects of DNA replication timing on mutation rates. The figure shows the AIMF for regions residing within constant early (purple) and constant late DNA replication timing zones (orange) for completely sequenced genomes of five cancer types and two personal genomes: (a) melanoma of study 1 (1 sample)25, (b) melanoma of study 2 (25 samples in total)26, (c) prostate cancer (7 samples in total)27, (d) small cell lung cancer (1 sample)28, (e) chronic lymphocytic leukaemia (4 samples in total)29, (f) colorectal cancer (9 samples in total)30, (g) Watson31and (h) HuRef genomes32. The AIMF represents the number of SNS observed per base pair in the FIRs, which overlap with constant early and constant late DNA replication timing zones, respectively. The horizontal axes display the results for chr1–chr22 and chrX. Description of analysed data sets We integrated SNS data from completely sequenced genomes of five cancer types (melanoma [25] , [26] , prostate cancer [27] , small cell lung cancer [28] , chronic lymphocytic leukemia [29] and colorectal cancer [30] ; the number of samples analysed is shown in Table 1 ), two completely sequenced personal genomes [31] , [32] , genome-wide DNA replication timing data [23] , [24] and data on single-nucleotide differences between the human (hg18) and chimpanzee (panTro2) genomes [33] . All data were mapped to the human genome version hg18. Genome-wide replication timing data, obtained using a technique based on massively parallel sequencing (Repli-Seq) across different human cell types [23] , were used to classify genomic regions as ‘constant early’, ‘constant mid’, ‘constant late’ and ‘variable’, according to the extent of consistency of replication timing regions across the different cell types. Table 1 Cancer types and numbers of samples used in this study. Full size table Because cancer development encompasses two intertwined processes—the acquisition of mutations and natural selection affecting the frequency of the resultant phenotypes [3] , we first excluded regions such as the centromere and telomere, Y chromosome, genes and promoters (±2 kb), repeat elements and ultra-conserved regions [33] from the data. The remaining sequences were expected to evolve nearly neutrally and were termed filtered intergenic regions (FIRs). Using FIRs only, we were also able to avoid some challenging issues of variant calling outside of these regions [34] . The frequency of mutations detected in these regions was referred to as adjusted intergenic mutation frequency (AIMF). We mapped SNS data for each cancer genome onto the FIRs and calculated the AIMF for both the whole genome and each chromosome individually. 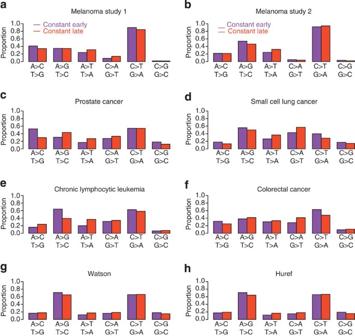Figure 2: Relationship between DNA replication timing and substitution patterns. The figure shows the proportions of different types of SNS in the constant early (purple) and constant late (orange) DNA replication timing zones for completely sequenced genomes of five cancer types and two personal genomes: (a) melanoma of study 125, (b) melanoma of study 226, (c) prostate cancer27, (d) small cell lung cancer28, (e) chronic lymphocytic leukaemia29, (f) colorectal cancer30, (g) Watson31and (h) HuRef genomes32. The proportions were calculated based on the hg18 reference allele so that Prob(A→C: T→G)+Prob(A→G: T→C)+Prob(A→T: T→A)=100%, and Prob(C→A: G→T)+Prob(C→T: G→A)+Prob(C→G: G→C)=100% for each of the constant late and constant early categories. Note that A→T: T→A is a signature commonly higher in late replication timing in all cancer types. Using theχ2-test and correcting for multiple hypothesis testing by false discovery rate,b,c,gandhare significantly different with adjustedP-values <0.01. Our analysis revealed that the AIMF varies substantially across the four cancer types ( Table 2 and Supplementary Table S1 , based on analysis of variance adjusted by multiple comparisons); such variation could be explained by biological differences in the cancer types and/or differences in the experimental design, sequencing technologies and variant calls. Nevertheless, similar trends were observed in the two completely sequenced personal genomes [31] , [32] , pointing towards meaningful differences ( Table 2 ). 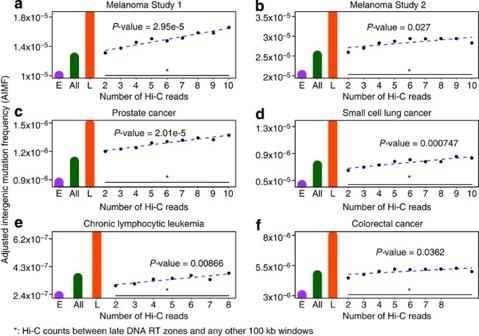Figure 3: Higher-order nuclear architecture is associated with mutation frequencies. The figure shows the AIMF in the ‘transition-to-late’ regions defined by different numbers of Hi-C interaction counts from the GM06990 cell line between regions inside and outside the constant late DNA replication timing zones for (a) the melanoma sample of study 125, (b) melanoma samples of study 226, (c) prostate cancer samples27, (d) the small cell lung cancer sample28, (e) chronic lymphocytic leukaemia samples29and (f) colorectal cancer samples30. Statistical significance was evaluated using simple linear regression, andP-values were obtained. AllP-values were <0.01. The green bar shows the genome-wide AIMF, the orange bar shows the AIMF in constant late DNA replication timing FIR and the purple bar shows the AIMF in constant early DNA replication timing FIR. The blue dashed line, that is, the fitted linear model, shows the positive association between the AIMF and the Hi-C counts that was used to stratify the regions. Because of the small mutation number in the chronic lymphocytic leukaemia genome, we only used 2–8 Hi-C counts ind. The x-axes display the groups of regions stratified by the number of Hi-C interactions with constant late replication timing regions. We then also repeated these analyses using genome-wide data instead of FIRs and obtained consistent results ( Table 3 ). Table 2 The genome-wide AIMF. Full size table Table 3 The genome-wide mutation frequency (MF). Full size table Mutation frequencies depend on replication timing We first sought to investigate the effects of DNA replication timing onto the patterns of SNS frequency in cancer genomes. We utilized only constant late and constant early replication timing zones [23] to exclude tissue specificity as a confounding factor. The constant mid category represented a much smaller part of the human genome and was thus discarded. We first analysed the melanoma genomes [25] . We observed that the mutation frequency in the FIRs was intimately linked to DNA replication timing: FIRs with constant late replication timing displayed a significantly higher AIMF compared with those with constant early replication timing (Mann–Whitney U -test P- value=2.075 × 10 −7 ). This effect was consistent across all 23 chromosomes (chr1-22 and chrX). We did not identify a significant trend when investigating the 23 chromosomes individually ( Fig. 1 and Supplementary Figs S1–S13 ). We then repeated our analysis for the other four cancer types (prostate cancer, small cell lung cancer, chronic lymphocytic leukaemia and colorectal cancer) and two personal genomes (Watson [31] and HuRef [32] genomes, analysed separately) and obtained similar results ( Fig. 1 ). Using a permutation test based on randomly permuting the number of mutations in the adjusted intergenic regions ( Supplementary Figs S14 and S15 ), we recalculated the permuted AIMFs and compared them with the observed patterns, obtaining a permutation P- value <0.001 for all cancer types. To investigate the confounding effects of different genomic features, we then adjusted for a variety of potential confounders such as gene density, GC percentage, recombination rate, CpG islands, chromatin states [9] and nuclear lamina-associated regions [11] ( Supplementary Figs S1–S13 and Table 2 ). The observed patterns of SNS with regard to replication timing were consistent in different groups categorized by these genomic features for all analysed genomes. This observation suggests that our findings are unlikely biased by these genomic features and the internal biological variation among cancer types. Figure 1: Effects of DNA replication timing on mutation rates. The figure shows the AIMF for regions residing within constant early (purple) and constant late DNA replication timing zones (orange) for completely sequenced genomes of five cancer types and two personal genomes: ( a ) melanoma of study 1 (1 sample) [25] , ( b ) melanoma of study 2 (25 samples in total) [26] , ( c ) prostate cancer (7 samples in total) [27] , ( d ) small cell lung cancer (1 sample) [28] , ( e ) chronic lymphocytic leukaemia (4 samples in total) [29] , ( f ) colorectal cancer (9 samples in total) [30] , ( g ) Watson [31] and ( h ) HuRef genomes [32] . The AIMF represents the number of SNS observed per base pair in the FIRs, which overlap with constant early and constant late DNA replication timing zones, respectively. The horizontal axes display the results for chr1–chr22 and chrX. Full size image We then repeated our analyses using genome-wide mutation frequencies in constant late and constant early replication timing regions ( Table 3 ). In general, we obtained robust results. Surprisingly, in prostate cancer and small cell lung cancer, the genome-wide mutation frequencies were higher than the AIMF ( Tables 2 and 3 ); these findings might arise because of an excess of mutations in repeat elements in these two cancer types, which could be due to mapping issues, different criteria used for variant calls or diverse biological mechanisms of tumorigenesis. After adjusting for several genomic features, we again obtained results consistent with previous studies showing that genomic regions, which (i) have a high gene density, (ii) reside in euchromatin regions or (iii) have a high CpG content, display lower mutation rates. When analysing adjusted intergenic regions instead of the whole genome, however, some of these associations were not observed: for instance, we observed a relatively higher AIMF in melanoma samples as well as the Watson and HuRef genomes in regions with higher CpG density compared with lower CpG density. One possible reason for this observation is that SNS in FIRs might not be strongly affected by the active elements around the regions. Alternatively, this trend might also be because of sequencing or mapping issues in repeat elements. We also calculated the SNS frequencies in genes only: the SNS frequency in genes was much lower than the AIMF ( χ 2 -test, P- value <0.0001), and constant late replication timing regions had larger SNS frequencies in genes ( Supplementary Table S2 ). To account for the potential inconsistencies of replication timing across cell lines, we used six alternative replication timing data sets [24] , [35] , [36] from the Replication Domain database to confirm our findings ( Supplementary Fig. S16 ). Recent evidence suggests that DNA replication timing may be coordinated across megabase-scale domains in metazoan genomes, and that early and late replication initiation occurs in spatio-temporally separate nuclear compartments [13] , [14] , [19] . Thus, it is possible that DNA replication timing domains within a larger genomic region (for example, 1 Mb) might affect the SNS frequency. For instance, overall, constant late genomic material could reside in regions that are either predominantly replicated late or not, and vice versa. To address this issue, we segmented the human genome into 1 Mb non-overlapping windows and dichotomized these windows into those with a large versus small proportion of late-replicating domains based on the prevalence of late-replicating base pairs within them. Using different cutoffs to categorize these 1 Mb windows, we found that in the stratum with a large proportion of late RT material, the SNS frequencies are higher than in the stratum with a small proportion of late RT material ( χ 2 -test, P- value <0.001 in all cases), but the differences of mutation frequencies between specific early and late replication timing regions hold in both strata ( Supplementary Fig. S17 ). This observation was also consistent across the five cancer types. Therefore, the prevalence of late replication timing zones on a larger scale is unlikely to affect our observations. Interestingly, although it has been reported that the transition regions between late and early replication timing zones are less stable than other parts of the genome [37] , we did not observe significant differences in terms of mutation rates between regions at the centre versus at the boundary of individual replication timing zones based on the constant late and early replication timing data ( Supplementary Fig. S18 ). Different temporal phases of DNA replication have been reported to associate with the existence of DNA secondary structures [38] , common fragile sites [39] and sometimes cis -regulatory elements [40] . To examine whether these factors could confound the different mutation frequencies in early and late replication timing zones, stratification analyses were performed based on these factors ( Supplementary Fig. S19 ). The preference of SNS in constant late over constant early DNA replication timing was not masked by these factors, demonstrating remarkable robustness of our observation, in addition to other control analyses. Besides, we focused on intergenic mutations, whose function is difficult to be inferred computationally or verified experimentally [41] . However, some portion of the intergenic regions can potentially be transcribed [42] ; for instance, noncoding RNAs, especially large intergenic noncoding RNAs (lincRNAs), may also contribute to the local variation of the distribution of mutation frequencies [41] . A recent study has catalogued all known lincRNAs with the most thorough annotation to date [43] . Because those adjusted intergenic mutations included in our study are far away from protein-coding genes (median distance to the closest transcription start site: 400 kb), it is possible that these mutations have a role in acting on those lincRNAs. We observed that the SNS did not display any global preference towards residing within FIR regions overlapping with lincRNAs ( Supplementary Table S3 ). However, because we cannot rule out that mutations varying lincRNAs are more frequent in cancer genomes and the effects of variation in lincRNAs may be subtle compared with variation in protein-coding genes, more work is required to delineate these effects. Mutation signatures depend on replication timing When investigating the different types of SNS in cancer FIRs, we observed that the patterns depended on whether FIRs were located in constant early versus constant late replication timing zones. We considered six types of SNS signatures for each nucleotide in the genome: A→C: T→G, A→G: T→C, A→T: T→A, C→A: G→T, C→T: G→A and C→G: G→C. The proportions of these six types of substitutions were calculated for the constant late and constant early replication timing FIRs ( Fig. 2 ). The overall patterns were significantly different between constant early and constant late replication timing ( χ 2 -test, P- values <0.01 in all cases, Fig. 2 ). Similar differences of substitution patterns between early and late replication timing zones were obtained after controlling for the effects of gene density, GC percentage, chromatin state, CpG islands, recombination rate and nuclear lamina-associated regions ( Supplementary Figs S20–S31 ). Interestingly, we also obtained a similar trend using the single-nucleotide polymorphism data from the two completely sequenced personal genomes ( Fig. 2 and Supplementary Figs S20–S31 ). The mutation signatures within genes and promoters were also investigated ( Supplementary Fig. S32 ) to allow a comparison between genic and intergenic regions. We found similar patterns in genes and FIRs in terms of mutation signatures ( Supplementary Fig. S32 ). Figure 2: Relationship between DNA replication timing and substitution patterns. The figure shows the proportions of different types of SNS in the constant early (purple) and constant late (orange) DNA replication timing zones for completely sequenced genomes of five cancer types and two personal genomes: ( a ) melanoma of study 1 [25] , ( b ) melanoma of study 2 [26] , ( c ) prostate cancer [27] , ( d ) small cell lung cancer [28] , ( e ) chronic lymphocytic leukaemia [29] , ( f ) colorectal cancer [30] , ( g ) Watson [31] and ( h ) HuRef genomes [32] . The proportions were calculated based on the hg18 reference allele so that Prob(A→C: T→G)+Prob(A→G: T→C)+Prob(A→T: T→A)=100%, and Prob(C→A: G→T)+Prob(C→T: G→A)+Prob(C→G: G→C)=100% for each of the constant late and constant early categories. Note that A→T: T→A is a signature commonly higher in late replication timing in all cancer types. Using the χ 2 -test and correcting for multiple hypothesis testing by false discovery rate, b , c , g and h are significantly different with adjusted P- values <0.01. Full size image Comparing the data across cancer types, we observed some common patterns: some signatures were more prevalent in the constant late regions, whereas others were preferentially located in constant early regions. For instance, A→T: T→A transversions occurred most often in the constant late replication timing regions in all five cancer types. Out of the five cancer types and the two personal genomes studied, the differences of the proportion of A→T: T→A in early and late replication timing regions were significant in prostate cancer samples, melanoma samples from study 2, and Watson and HuRef genomes (adjusted P- values <0.01 after multiple testing correction). Overall, the higher proportion of A→T: T→A in late replication timing zones was observed in 38 out of all the 47 samples analysed in our study ( Supplementary Figs S33–S40 ). In contrast, the frequencies of mutations and the relative proportions of the six types of substitution signatures differed among the five cancer genomes and two personal genomes; for example, the most frequent type of substitution in melanoma was the C→T transition [25] . In general, the consistency in the relative proportions of substitution signatures in constant early versus constant late replication timing regions might indicate common mutagenic mechanisms in different temporal phases of DNA replication. Mutation frequencies and higher-order nuclear organization The spatio-temporal segregation of DNA replication timing leads to the formation of DNA replication factories in which DNA synthesis takes place on multiple strands simultaneously [13] , [14] . We therefore aimed to test the hypothesis that those regions brought in close spatial proximity by the proposed fractal organization of the genome [12] display similar mutation frequencies. To address this question, we divided the whole genome into 100 Kb non-overlapping windows and obtained Hi-C-based long-range interaction data from the GM06990 and K562 cell lines from Lieberman-Aiden et al . [12] to measure the spatial proximity between two individual windows. We excluded any two loci that were closer than 20 Kb from each other on linear DNA. We then stratified all pairs of windows according to the number of Hi-C reads between them and investigated those windows close to but outside of the constant late DNA replication timing zones. Those regions that overlapped with FIRs were referred to as ‘transition-to-late’ regions; these are the regions that do not reside in constant late replication timing zones but are linked to constant late regions with at least one Hi-C read. Compared with the AIMF in constant late and constant early DNA replication timing zones, we found that the AIMF in the ‘transition-to-late’ regions were much closer to, yet still smaller than that in constant late DNA replication timing zones. Interestingly, the AIMF was positively associated with the interaction counts (linear regression P- value <0.01 for each cancer type, Fig. 3 ). Furthermore, in most cases, the AIMF in these regions was higher than the genome-wide AIMF ( Fig. 3 ). These observations were consistent across the Hi-C data from the GM06990 and K562 cell lines and the Hi-C data for the GM06990 cell line generated using different restriction enzymes ( Hin dIII and Nco I) ( Supplementary Figs S41–S43 ). Figure 3: Higher-order nuclear architecture is associated with mutation frequencies. The figure shows the AIMF in the ‘transition-to-late’ regions defined by different numbers of Hi-C interaction counts from the GM06990 cell line between regions inside and outside the constant late DNA replication timing zones for ( a ) the melanoma sample of study 1 [25] , ( b ) melanoma samples of study 2 [26] , ( c ) prostate cancer samples [27] , ( d ) the small cell lung cancer sample [28] , ( e ) chronic lymphocytic leukaemia samples [29] and ( f ) colorectal cancer samples [30] . Statistical significance was evaluated using simple linear regression, and P- values were obtained. All P- values were <0.01. The green bar shows the genome-wide AIMF, the orange bar shows the AIMF in constant late DNA replication timing FIR and the purple bar shows the AIMF in constant early DNA replication timing FIR. The blue dashed line, that is, the fitted linear model, shows the positive association between the AIMF and the Hi-C counts that was used to stratify the regions. Because of the small mutation number in the chronic lymphocytic leukaemia genome, we only used 2–8 Hi-C counts in d . The x-axes display the groups of regions stratified by the number of Hi-C interactions with constant late replication timing regions. Full size image We also examined whether the different proportions of DNA replication timing (including constant early, constant mid, constant late and variable) in the transition zones confounded our results. To address this issue, we performed the following analysis: the FIRs were divided into four groups—(i) constant late regions linked with Hi-C reads to constant late regions, (ii) constant late regions linked with Hi-C reads to constant early regions, (iii) constant early regions linked with Hi-C reads to constant late regions and (iv) constant early regions linked with Hi-C reads to constant early regions. We found that group (i) had the highest mutation frequency, whereas group (iv) had the lowest. Moreover, the mutation frequency of group (ii) was closer to, but still lower than that of group (i), and a similar trend was observed between groups (iii) and (iv) ( Fig. 4 ). Interestingly, all pairwise comparisons were significantly different (Mann–Whitney U -test, false discovery rate-adjusted P- value <0.03 in all cases). Taken together, we found that those regions close to late DNA replication timing zones had similar, though lower, mutation frequencies, suggesting a potential role for higher-order chromatin organization on the mutagenic mechanisms during DNA replication. 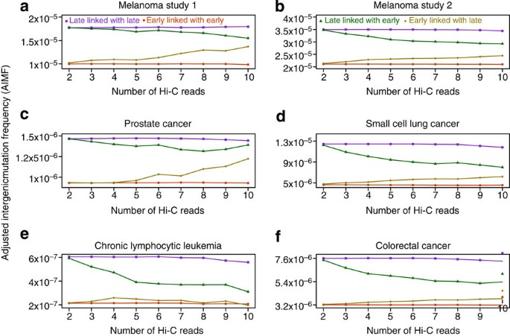Figure 4: Effects of transition regions on mutation frequencies. The figure shows the AIMF for (a) the melanoma sample of study 125, (b) melanoma samples of study 226, (c) prostate cancer samples27, (d) the small cell lung cancer sample28, (e) chronic lymphocytic leukaemia samples29and (f) colorectal cancer samples30in four groups of adjusted intergenic regions: constant late replication timing regions linked with constant late replication timing regions by Hi-C interactions (purple); constant late replication timing regions linked with constant early replication timing regions by Hi-C interactions (green); constant early replication timing regions linked with constant late replication timing regions by Hi-C interactions (gold); and constant early replication timing regions linked with constant early replication timing regions by Hi-C interactions (red). The x-axes display the groups of paired regions stratified by the number of Hi-C reads (2–10). All pairwise comparisons were significantly different from each other (Mann–WhitneyU-test, false discovery rate-adjustedP-values <0.03 in all cases). Figure 4: Effects of transition regions on mutation frequencies. The figure shows the AIMF for ( a ) the melanoma sample of study 1 [25] , ( b ) melanoma samples of study 2 [26] , ( c ) prostate cancer samples [27] , ( d ) the small cell lung cancer sample [28] , ( e ) chronic lymphocytic leukaemia samples [29] and ( f ) colorectal cancer samples [30] in four groups of adjusted intergenic regions: constant late replication timing regions linked with constant late replication timing regions by Hi-C interactions (purple); constant late replication timing regions linked with constant early replication timing regions by Hi-C interactions (green); constant early replication timing regions linked with constant late replication timing regions by Hi-C interactions (gold); and constant early replication timing regions linked with constant early replication timing regions by Hi-C interactions (red). The x-axes display the groups of paired regions stratified by the number of Hi-C reads (2–10). All pairwise comparisons were significantly different from each other (Mann–Whitney U -test, false discovery rate-adjusted P- values <0.03 in all cases). Full size image Evolutionary and cancer mutations share genomic locations We then sought to compare the regions prone to accumulating adjusted intergenic SNS in cancer genomes versus mutations arising on evolutionary time scales. To this end, we obtained data on differences between the human hg18 and chimpanzee panTro2 genomes from the UCSC genome browser [33] , using a similar approach as in Stamatoyannopoulos et al ., [18] and compared the number of such changes with the number of SNS in each cancer type in 1 Mb non-overlapping windows [44] . The five cancer types had very different regions that overlapped with those regions harbouring human–chimpanzee SNS ( Supplementary Fig. S44 ). After collapsing the windows with SNS in each of the five cancer types together, we identified 1,039 such windows with at least one SNS in any of the five cancer types in early DNA replication timing zones. We then fixed the number of windows with cancer mutations and selected the same number of windows with the highest number of human–chimpanzee SNS. Out of these 1,039 windows, 775 were also present among the human–chimpanzee SNS windows. We then performed similar analyses in late DNA replication timing zones and found that out of 1,240 windows, 1,208 overlapped in cancer and human–chimpanzee SNS ( Supplementary Fig. S45 ). Although the overlap between regions with cancer SNS and the regions with the top human–chimpanzee SNS varied across different cancer types, after pooling them together, the overlap became larger. Therefore, we concluded that at the scale of 1 Mb, most regions harbouring human–chimpanzee SNS were also regions harbouring SNS in any one of the five cancer types. This finding suggests some common mechanisms between human–chimpanzee evolutionary transversion and cancer mutagenesis, with no obvious differences in early versus late DNA replication timing zones. In this paper, we have demonstrated that mutational landscapes of cancer genomes differ between early and late DNA replication timing zones, with higher mutation frequencies in late replication timing regions. We identified different patterns of mutation signatures across these zones; for example, A→T: T→A mutation signatures commonly appeared in most cancer samples investigated. This finding implies that some mutagenic and repair mechanisms might depend on the DNA replication timing of genomic material. The differences in mutation frequencies and signatures between early and late replication timing also hold after controlling for several genomic features such as GC percentage, CpG density, recombination rate, chromatin accessibility, gene density and lamina-associated domains. Also, the transition-to-late regions defined based on Hi-C interactions, although not located in constant late replication timing regions, has higher mutation frequencies than the overall AIMF. Taken together, we conclude that (i) DNA replication timing is a robust genomic feature affecting SNS frequencies in both cancer and personal genomes, after controlling for many variables such as GC percentage, gene density, recombination rate, higher-order DNA replication timing domains, CTCF-binding sites, secondary structures and lincRNAs; (ii) SNS display specific patterns in early versus late DNA replication timing regions; and (iii) higher-order nuclear organization, together with DNA replication timing, affects the mutation frequencies. Furthermore, we found that in general, genome-wide mutation frequencies were lower than AIMFs. The exceptions in prostate cancer and small cell lung cancer could be because of an excess of mutations in repeat elements observed in our analysis, because the majority of the regions excluded from the genome to determine the AIMF were genes, promoters and repeat elements. The overall higher genome-wide mutation frequency in late replication timing regions also holds after controlling for several genomic features. The higher SNS frequencies in late DNA replication timing zones in cancer genomes could partly arise from the accumulation of single-stranded DNAs, given similar observations in our analyses and others [18] and given that a certain fraction of regions harbouring mutations overlapped between cancer and personal genomes ( Supplementary Fig. S45 ). DNA repair processes can often repair the errors arising during replication [45] , and it has been suggested that both DNA replication timing and the efficiency of DNA repair are related to higher-order chromatin structure [45] , [46] . Our findings suggest that some portions of the genome have similar mutation frequencies as their counterparts residing closely within the three-dimensional structure of the nucleus. Chromatin organization and replication timing are intertwined, and could be a driving force of carcinogenesis by disrupting specific processes such as replication initiation and replication fork progression [46] . However, because most mutations analysed reside in noncoding parts of the genome, these patterns might only have indirect applicability to an understanding of the origins of cancer. Our study represents a novel approach to study the replication process-related SNS in cancer genomes together with the higher-order nuclear organization of the genome. This approach can lead to a better understanding of the mutational landscape of cancer genomes from the perspective of replication, epigenetics and chromatin structure. Data sets and analyses Cancer types and sample numbers analysed are listed in Table 1 . All analyses were performed using human genome version hg18 as the reference genome. To obtain the FIRs, we employed a similar approach as was used by two other studies [18] , [47] . We removed all Refseq genes and promoters (up to 2 kb upstream of a gene), ultra-conserved elements with a conservation score >300 and also intronic sequences, which are related to transcription-coupled DNA repair. We also excluded repeat elements, centromeres and telomeres to minimize variant calling complexity in these regions [48] , as well as the Y chromosome. All of these data were downloaded from the UCSC genome browser from the NCBI36/hg18 human genome [49] . The remaining genomic regions were termed FIRs. The total length of FIRs was approximately 780 Mb. We then overlaid the DNA replication timing data obtained from Hansen et al . [23] onto the FIRs and found that 79.23 Mb and 169.50 Mb of the FIRs resided within replicating regions that were consistently early or late, respectively, across multiple cell types. The human GC percentage, CpG island and recombination rate data were also obtained from UCSC genome browser. Because highly compact heterochromatin stains for Giemsa, whereas euchromatin is often unstained, we were able to characterize euchromatin and heterochromatin states globally across different cell types using Giemsa staining data [50] . Data on nuclear lamina-associated domains from Guelen et al . [11] were obtained from the NCBI Gene Expression Omnibus database, accession code GSE8854. Genomic regions harbouring nuclear lamina-associated domains are referred to as the nuclear periphery, whereas the remaining regions are referred to as nuclear core. When analysing the effects of lamina-associated domains on the mutation patterns, we used a bootstrap sampling approach ( Supplementary Fig. S13 ) to take into account the variability of nuclear topology across different cell types. The Hi-C data for GM06990 and K562 cell lines were obtained from Lieberman-Aiden et al . [12] through the Gene Expression Omnibus database. Moreover, data on genome-wide common fragile sites were obtained from Durkin and Glover. [39] The G-quadruplex and CTCF-binding site locations were obtained from Quadruplex.org [51] and CTCFBSDB [52] , respectively. The lincRNA catalogue can be obtained from http://www.broadinstitute.org/genome_bio/human_lincrnas [43] . All statistical calculations were performed using open source R software. When necessary, ‘liftover’ software was used to map data from other human genome versions to hg18. How to cite this article: Liu L et al . DNA replication timing and higher-order nuclear organization determine single-nucleotide substitution patterns in cancer genomes. Nat. Commun. 4:1502 doi: 10.1038/ncomms2502 (2013).